Hierarchically porous carbons with optimized nitrogen doping as highly active electrocatalysts for oxygen reduction Development of efficient, low-cost and stable electrocatalysts as the alternative to platinum for the oxygen reduction reaction is of significance for many important electrochemical devices, such as fuel cells, metal–air batteries and chlor-alkali electrolysers. Here we report a highly active nitrogen-doped, carbon-based, metal-free oxygen reduction reaction electrocatalyst, prepared by a hard-templating synthesis, for which nitrogen-enriched aromatic polymers and colloidal silica are used as precursor and template, respectively, followed by ammonia activation. Our protocol allows for the simultaneous optimization of both porous structures and surface functionalities of nitrogen-doped carbons. Accordingly, the prepared catalysts show the highest oxygen reduction reaction activity (half-wave potential of 0.85 V versus reversible hydrogen electrode with a low loading of 0.1 mg cm −2 ) in alkaline media among all reported metal-free catalysts. Significantly, when used for constructing the air electrode of zinc–air battery, our metal-free catalyst outperforms the state-of the-art platinum-based catalyst. Electrochemical oxygen reduction is a critical process for many energy storage and conversion devices that operate in acidic (for example, proton exchange membrane fuel cells) or basic electrolytes (for example, alkaline fuel cells, metal–air batteries, chlor-alkali electrolysers, and so on). Developing active and durable oxygen reduction reaction (ORR) electrocatalysts is crucial for successful implementation of these technologies. Although Pt and Pt-based alloys have proven to be the most efficient catalysts for ORR, the prohibitive cost and scarcity of Pt-based catalysts significantly hinder their large-scale applications [1] , [2] . An additional drawback associated with Pt is the poor durability caused by different degradation mechanisms during long-term electrochemical operation, such as nanoparticle migration, Ostwald ripening, coalescence and leaching [3] , [4] , [5] . Great efforts have been devoted to search for efficient, durable and inexpensive alternatives to Pt-based ORR catalysts [6] , [7] , [8] , [9] , [10] , [11] , [12] , [13] , [14] , [15] , [16] , [17] . Nitrogen-doped nanostructured carbon materials represent important candidates as metal-free electrocatalysts for ORR because of their unique electronic properties and structural features [18] , [19] , [20] . In spite of some significant achievements attained by the careful selection of suitable precursors and the optimization of nanostructuring process [18] , [21] , [22] , [23] , [24] , [25] , [26] , [27] , [28] , the ORR performance of the reported metal-free catalysts is still inferior to the state-of-the-art Pt/C catalyst in terms of half-wave potential and does not yet warrant implementation in real energy conversion/storage devices. To make metal-free catalysts truly competitive with Pt/C, two crucial factors that govern the performance of the carbon-based, metal-free ORR electrocatalysts have to be considered simultaneously: surface functionalities (mainly the doped nitrogen content and type), which determine the intrinsic nature of active sites, namely the turnover frequency (TOF) per active site, and specific surface area and porous structure. Regarding the TOF, it is believed that the nitrogen types and ratios are crucial for ORR, albeit an in-depth understanding is still required. On the other hand, a hierarchically porous structure, in particular, with a meso/micro multimodal pore size distribution (PSD), is highly desirable for ORR, as high microporosity can supply numerous accessible active sites, while rich mesoporosity is favourable for the efficient mass transport in the catalyst layer [11] . Here we demonstrate the fabrication of nitrogen-doped metal-free ORR catalysts based on the combination of hard-templating synthesis with nitrogen-enriched aromatic polymers as precursors and NH 3 activation, targeting simultaneous optimization of both porous structures and surface functionalities of the catalysts. The prepared catalysts possess a high specific surface area of 1,280 m 2 g −1 , a hierarchically porous structure with meso/micro multimodal PSD, and an optimized surface functionality with the desired nitrogen doping. These unique structural features lead to the highest ORR activity (half-wave potential of 0.85 V versus reversible hydrogen electrode (RHE) with a low loading of 0.1 mg cm −2 ) in alkaline media among all reported nitrogen-doped carbon catalysts [18] , [21] , [22] , [23] , [24] , [25] , [26] , [27] , [28] . Furthermore, the full-cell (Zn–air battery) performance of the prepared catalyst outperforms the state-of the-art Pt/C catalyst (20 wt% Pt, BASF). These results clearly reveal that the developed metal-free catalyst promises to replace Pt-based noble metal catalysts for many important electrochemical devices, including metal–air batteries, alkaline fuel cells and chlor-alkali electrolysers. Electrocatalyst synthesis The fabrication of hierarchically porous catalysts was based on the hard-templating synthesis combined with NH 3 activation, as illustrated in Fig. 1 . Mesoporous nitrogen-doped carbon (denoted as meso-P o PD) was first prepared through the polymerization of o -phenylenediamine ( o PD) in the presence of silica colloid followed by the pyrolysis of P o PD/silica composite at 900 °C under flowing argon and final NaOH (2 M) etching. The aromatic feature and high N/C atomic ratio (=0.34) for P o PD allow for the production of doped carbons with a high nitrogen content of 9.5 at%. The prepared meso-P o PD was then subjected to a second heat treatment under NH 3 to further enhance the porosity, resulting in the hierarchically porous N-doped carbon (denoted as meso/micro-P o PD). For comparison, N-doped carbon with low porosity (denoted as p-P o PD) was prepared by direct pyrolysis of P o PD without silica colloid. Microporous nitrogen-doped carbon (denoted as micro-P o PD) was prepared by activation of p-P o PD with NH 3 . 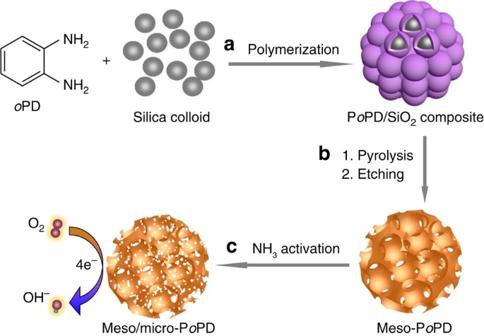Figure 1: Schematic illustration of the synthesis of meso/micro-PoPD electrocatalyst. (a) Polymerization ofoPD in the presence of silica colloid by addition of ammonium peroxydisulphate (APS). (b) Pyrolysis of PoPD/SiO2nanocomposite in N2atmosphere and subsequent etching of the SiO2template with 2.0 M NaOH solution to yield meso-PoPD. (c) Further activation of the meso-PoPD with NH3and formation of the final meso/micro-PoPD catalyst. The fabrication details and denotation of all samples in this work were summarized in Supplementary Table 1 . Figure 1: Schematic illustration of the synthesis of meso/micro-P o PD electrocatalyst. ( a ) Polymerization of o PD in the presence of silica colloid by addition of ammonium peroxydisulphate (APS). ( b ) Pyrolysis of P o PD/SiO 2 nanocomposite in N 2 atmosphere and subsequent etching of the SiO 2 template with 2.0 M NaOH solution to yield meso-P o PD. ( c ) Further activation of the meso-P o PD with NH 3 and formation of the final meso/micro-P o PD catalyst. Full size image Electrocatalyst characterization Transmission electron microscopy (TEM) revealed that the meso-P o PD consisted of a three-dimensional disordered pore system of spherical pores with an average diameter of ca. 15 nm and a shell thickness of 1–3 nm ( Fig. 2a and Supplementary Fig. 1 ), exactly reflecting the geometric characteristics of a silica sphere packing in the polymer/carbon-based composites ( Fig. 1 ). The well-defined mesoporous feature of meso-P o PD survived well after NH 3 activation at high temperature ( Fig. 2b and Supplementary Fig. 1 ). 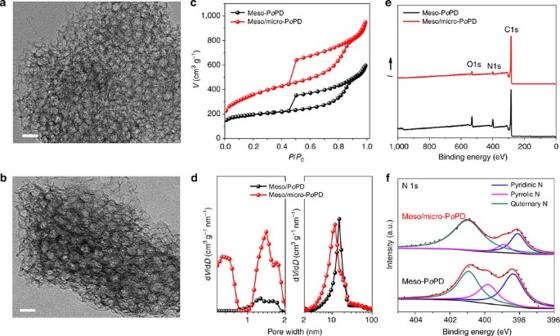Figure 2: Structural and compositional characterization of meso/micro-PoPD catalyst. (a,b) TEM images of meso-PoPD (a) and meso/micro-PoPD (b), showing the highly porous structures. Scale bars, 30 nm. (c) N2adsorption/desorption isotherms of meso-PoPD and meso/micro-PoPD. (d) The corresponding pore size distribution curves calculated from the adsorption branches. (e) X-ray photoelectron spectroscopy (XPS) survey spectra of meso-PoPD and meso/micro-PoPD catalysts. (f) High-resolution N 1s spectra of meso-PoPD and meso/micro-PoPD catalysts. N 2 adsorption–desorption tests were performed to evaluate the textural properties of the carbons and the results were summarized in Supplementary Table 2 . Both meso-P o PD and meso/micro-P o PD exhibited type-IV isotherm characteristics for mesoporous materials ( Fig. 2c ). The steep and high capillary condensation steps revealed uniform and well-developed mesoporosity with large mesopore volume, which is consistent with the TEM observations. After NH 3 activation, the Barrett–Emmett–Teller (BET) surface area increased dramatically from 685 m 2 g −1 for meso-P o PD to 1,280 m 2 g −1 for meso/micro-P o PD without substantial deterioration of mesoporosity ( Fig. 2c , Supplementary Table 2 ). Notably, the surface area of the meso/micro-P o PD originated from both mesopores ( S mesopore , 751 m 2 g −1 ) and micropore ( S micropore , 515 m 2 g −1 ). The PSD plots indicated that the meso/micro-P o PD possessed ultramicropore, micropore and mesopore centred at 0.6, 1.4 and 12 nm, respectively ( Fig. 2d ), further confirming the hierarchical porous structure in which micropores were incorporated into the walls of well-defined mesopores. The p-P o PD prepared without using a silica colloid template showed a low S BET of only 40 m 2 g −1 , which increased to 277 m 2 g −1 after NH 3 activation for micro-P o PD with major contribution from the micropores ( Supplementary Table 2 ). Figure 2: Structural and compositional characterization of meso/micro-P o PD catalyst. ( a , b ) TEM images of meso-P o PD ( a ) and meso/micro-P o PD ( b ), showing the highly porous structures. Scale bars, 30 nm. ( c ) N 2 adsorption/desorption isotherms of meso-P o PD and meso/micro-P o PD. ( d ) The corresponding pore size distribution curves calculated from the adsorption branches. ( e ) X-ray photoelectron spectroscopy (XPS) survey spectra of meso-P o PD and meso/micro-P o PD catalysts. ( f ) High-resolution N 1s spectra of meso-P o PD and meso/micro-P o PD catalysts. Full size image X-ray photoelectron spectroscopy measurements were performed to analyse the changes of surface functionalities of meso-P o PD during NH 3 activation. Most oxygen-containing groups that come from the oxygen implantation by the SiO 2 template were removed during NH 3 activation ( Fig. 2e ). This can be explained by the reactions between NH 3 and oxygen functionalities located on the carbon surface, possibly resulting in new nitrogen-containing active sites [12] , [29] . Surprisingly, the final nitrogen content of meso/micro-P o PD (3.15 at%) obtained with NH 3 activation was significantly lower than that of meso-P o PD (9.5 at%), although NH 3 was generally recognized as a nitrogen precursor for preparing N-doped carbon catalysts [10] , [11] , [12] , [18] , [19] . We reason that, besides the surface reaction with oxygen species, NH 3 molecules can also react with the carbon matrix under high temperature, preferably with disordered carbon phases [30] , [31] , [32] . Such an etching reaction process would burn off carbon significantly together with elimination of nitrogen moieties that originate from the nitrogen-enriched polymers. Interestingly, the relative amount of quaternary nitrogen increased with NH 3 activation from 38% for meso-P o PD to 71% for meso-micro-P o PD ( Fig. 2f ). Although the details of the surface chemistry occurring during NH 3 activation remain elusive, these results clearly suggest that the NH 3 activation not merely improve the porosity of meso-P o PD but also dramatically restructures its surface functionalities, both of which are crucial for enhancing the ORR activity. Electrocatalytic performance We performed cyclic voltammetry and rotating disk electrode (RDE) measurements in 0.1 M KOH to evaluate the ORR activity of meso/micro-PoPD catalyst and several reference P o PD-derived carbon materials (p-P o PD, micro-P o PD and meso-P o PD). A state-of-the-art commercial Pt/C catalyst (20% Pt, BASF) was also measured under the same conditions for comparison. Cyclic voltammetry measurements in O 2 -saturated electrolyte showed that the peak potential at 0.83 V versus the RHE afforded by meso/micro-P o PD catalyst was comparable to that of Pt/C (0.84 V), but much higher than that of other control samples (0.56, 0.67 and 0.76 V for p-P o PD, micro-P o PD and meso-P o PD, respectively, Supplementary Fig. 2 ). The high ORR activity of the meso/micro-P o PD catalyst was further confirmed by the RDE measurements ( Fig. 3a ). The p-P o PD with low porosity exhibited poor electrocatalytic activity with a large ORR overpotential, attributable to the low density of active sites exposed to electrochemical interface. Either NH 3 activation for preparing the micro-P o PD or templating synthesis for preparing the meso-P o PD could create N-doped carbon materials with improved porosity and thus enhance the ORR activity when compared with p-P o PD. Particularly, the hierarchically porous meso/micro-P o PD catalyst exhibited substantial improvement in ORR activity, as reflected by the shift of the half-wave ( E 1/2 ) potential to 0.85 V, well comparable to the Pt/C catalyst ( E 1/2 =0.85 V) with the same loading of 0.1 mg cm −2 ( Fig. 3b ). Considering the technical and economic feasibility, we increased the catalyst loading of meso/micro-P o PD to 0.5 mg cm −2 , yielding a further improved E 1/2 value of 0.87 V, which was 20 mV more positive than that of Pt/C catalyst ( Fig. 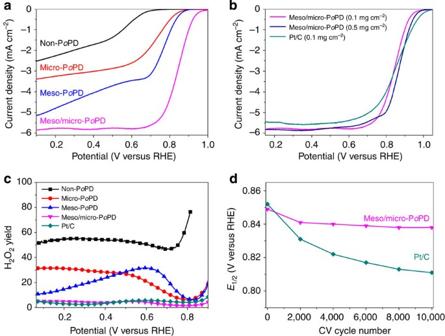Figure 3: Electrocatalytic performance of the catalysts. (a) ORR polarization plots of meso/micro-PoPD and reference catalysts. The loading was 0.1 mg cm−2for all materials. (b) ORR polarization plots of meso/micro-PoPD with low (0.1 mg cm−2) and high loading (0.5 mg cm−2) and Pt/C catalyst (20 wt% Pt, BASF, loading, 0.1 mgcatalystcm−2). (c) H2O2yields plots of meso/micro-PoPD, reference materials, and Pt/C catalyst. (d) Half-wave potential of meso/micro-PoPD and Pt/C with the same loading of 0.1 mg cm−2as a function of the number of potential cycles in O2-saturated electrolyte. RDE and RRDE were recorded in 0.1 M KOH. Electrode rotation speed, 1,600 r.p.m.; scan rate, 10 mV s−1. 3b ) and higher than all previously reported results for heteroatom-doped carbon metal-free catalysts ( Supplementary Table 3 ). As a metal-free catalyst, the meso/micro-P o PD also showed prominent ORR activity with an onset potential of 0.84 V in acidic media, although the activity is still inferior to the Pt/C catalyst ( Supplementary Fig. 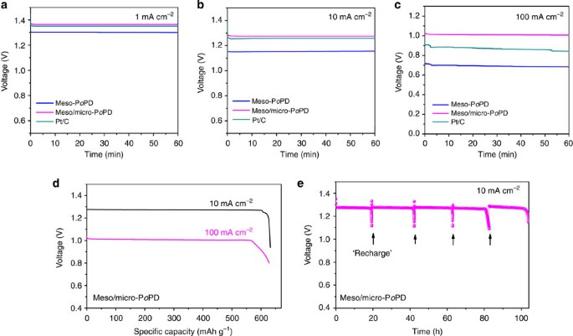Figure 4: Zn–air battery performance of the catalysts. (a–c) Typical galvanostatic discharge curves of Zn–air cells with meso-PoPD, meso/micro-PoPD and Pt/C as cathode catalysts at different current densities: (a) 1 mA cm−2, (b) 10 mA cm−2and (c) 100 mA cm−2. (d) Long-time galvanostatic discharge curves of Zn–air cell with meso/micro-PoPD as cathode catalyst until complete consumption of Zn anode. The specific capacity was normalized to the mass of consumed Zn. (e) ‘Recharging’ the Zn–air battery with meso/micro-PoPD as cathode catalyst by replenishing Zn anode and electrolyte. Electrolyte for Zn–air cell was 6.0 M KOH. Catalyst loading was 1.0 mg cm−2for all materials. The arrows indicate ‘recharging’ process. 3 and Supplementary Table 4 ). Figure 3: Electrocatalytic performance of the catalysts. ( a ) ORR polarization plots of meso/micro-P o PD and reference catalysts. The loading was 0.1 mg cm −2 for all materials. ( b ) ORR polarization plots of meso/micro-P o PD with low (0.1 mg cm −2 ) and high loading (0.5 mg cm −2 ) and Pt/C catalyst (20 wt% Pt, BASF, loading, 0.1 mg catalyst cm −2 ). ( c ) H 2 O 2 yields plots of meso/micro-P o PD, reference materials, and Pt/C catalyst. ( d ) Half-wave potential of meso/micro-P o PD and Pt/C with the same loading of 0.1 mg cm −2 as a function of the number of potential cycles in O 2 -saturated electrolyte. RDE and RRDE were recorded in 0.1 M KOH. Electrode rotation speed, 1,600 r.p.m. ; scan rate, 10 mV s −1 . Full size image When optimizing the P o PD-derived catalysts, it was found that the duration of NH 3 activation had a large influence on the ORR activity. The elemental compositions, texture properties, and ORR performance of a series of samples that were prepared by varying the NH 3 activation time were summarized in Supplementary Figs 4 and 5 and Supplementary Table 5 . We found that the ORR activity first grew fast with NH 3 activation duration and reached a plateau after 15 min. Such a trend is almost the same as that of weight-loss percentage and BET surface area with activation duration, validating a strong correlation between the ORR activity and the porosity of these catalysts. On the other hand, in contrast to the improved ORR activity with NH 3 activation, the total nitrogen contents decreased gradually, while the relative amount of quaternary nitrogen went up and achieved the maximum at 15 min ( Supplementary Table 5 ). These results suggest that the catalytic activity of P o PD-derived catalysts is also dependent on the proportion of doped quaternary nitrogen, instead of on the total amount of nitrogen species [33] . It is normally believed that pyridinic N doped at the edge of the graphitic layers is effective for ORR as such N-doping can reduce the energy barrier for oxygen adsorption on adjacent carbon atoms, and accelerate the rate-limiting first-electron transfer during the ORR [20] . Quantum theory calculation and previous experimental results also suggested that doping of quaternary N into graphene planes could induce a non-uniform electron distribution and short C–N bonds, comparable to O–O bonds, which would facilitate O 2 adsorption and subsequent disassociation/weakening of O=O bonds [19] , [21] . To further understand the origin of high activity of the catalysts, we performed the Koutecky–Levich (K-L) analysis to estimate the kinetic current densities of the catalysts within the mixed kinetic-diffusion controlled region and normalized them to the specific surface areas ( Supplementary Fig. 6 and Supplementary Note 1 ). Clearly, the performance gaps between different catalysts decreased obviously after normalization of kinetic current densities by the BET surface area ( Supplementary Fig. 6a,b ). After normalization, for example, the difference of the kinetic current densities between meso/micro-P o PD and meso-P o PD decreased from 10 to 5 times ( Supplementary Fig. 6c ). These results indicated that the increased specific surface area of meso/micro-PoPD contributed, but only partly, to the enhanced ORR activity. The intrinsic activity, namely the TOF per active site, would be another key factor governing the ORR activity of our catalysts. The electrochemical impedance spectroscopy measurements ( Supplementary Fig. 7 and Supplementary Note 2 ) revealed that the charge-transfer resistance of meso/micro-P o PD was much lower than those of other reference materials ( Supplementary Fig. 7a–c ), suggesting the faster kinetic process of oxygen reduction on meso/micro-P o PD catalysts compared with reference materials. Interestingly, the meso/micro-P o PD exhibited lower intrinsic resistance than meso-P o PD ( Supplementary Fig. 7d ), as result of the decrease in oxygen-containing groups after NH 3 activation ( Supplementary Table 2 ). The high proportion of doped quaternary nitrogen and improved conductivity probably lead to the enhanced intrinsic activity of meso/micro-PoPD. The rotating ring-disk electrode (RRDE) study revealed a high selectivity of the meso/micro-P o PD catalyst towards the four-electron reduction of oxygen ( Fig. 3c ). Even at a low loading of 0.1 mg cm −2 , the H 2 O 2 yield measured with meso/micro-P o PD remained below 5% at all potentials and dropped to 1.5% at 0.8 V, corresponding to a high electron-transfer number ( n e ) of 3.97. This value is much higher than that of p-P o PD, micro-P o PD and meso-PoPD ( n e =2.62–3.86), and slightly higher than that of Pt/C catalyst with n e of 3.92 at 0.8 V ( Fig. 3c and Supplementary Fig. 8 ). To evaluate the electrochemical durability of the catalysts, meso/micro-P o PD and Pt/C catalysts were cycled between 0.6 and 1.0 V at 50 mV s −1 in 0.1 M KOH under O 2 atmosphere. As shown in Fig. 3d and Supplementary Fig. 9 , very little change in half-wave potential (~10 mV) was observed for the meso/micro-P o PD even after 10,000 continuous potential cycles, while there was ~40 mV loss of half-wave potential for the Pt/C catalyst under the same condition, suggesting a superior durability of the meso/micro-P o PD catalyst. It is well known that commercial Pt/C catalysts suffer from nanoparticle migration, coalescence and even detaching from carbon supports during continuous electrochemical operation [1] , [3] , [5] , especially in the alkaline electrolytes used for alkaline fuel cells and metal–air batteries, which remains the major challenge for implementation of these technologies. In addition to the use of NH 3 , we also examined KOH and CO 2 as activation agents to prepare the highly porous catalysts based on the meso-P o PD. The obtained materials exhibited much lower ORR activity than meso/micro-P o PD in terms of onset/half-wave potentials and diffusion-limited current densities ( Supplementary Fig. 10 ), even though they had also high BET surface areas of 1,278–1,348 m 2 g −1 ( Supplementary Fig. 11 ) and considerable nitrogen-doping levels (5.68–5.90 at%) as well. Note that both KOH and CO 2 activation increased the amount of oxygen-containing groups greatly from 7.0 at% to 15.6–19.8 at%. The incorporation of abundant oxygen species would certainly introduce abundant defects on the carbon matrix and lead to reduced charge transport ability during eletrocatalysis ( Supplementary Fig. 7 ), which should be responsible for the low ORR activity of KOH/CO 2 -activated materials. On this basis, it is reasonable to conclude that NH 3 activation played a crucial role in achieving an optimal surface functionality of porous carbon catalysts for ORR. The present synthetic strategy can be generalized to produce highly active metal-free catalysts by using other nitrogen-enriched precursors, for example, polyaniline (PANI, N/C ratio=0.17), while keeping the fabrication procedure the same. Similar to meso/micro-P o PD, hierarchically porous structure with high BET surface area (1,190 m 2 g −1 ) and meso/micro PSD were also achieved for PANI-derived catalyst (meso/micro-PANI), as shown in Supplementary Figs 12 and 13 and Supplementary Table 2 . RDE polarization curves revealed the high ORR activity of meso/micro-PANI catalyst with a half-wave potential of 0.83 V, only slightly lower than that of meso/micro-P o PD ( Supplementary Fig. 14 ). In contrast, when sucrose (nitrogen-free) was used as precursor, the prepared material (meso/micro-sucrose) showed relatively poor electrocatalytic activity with a negative half-wave potential ( E 1/2 =0.77 V) and low diffusion-limited current density ( Supplementary Fig. 14 ), even though the NH 3 activation process introduced nitrogen doping for the meso/micro-sucrose (nitrogen content, 2.39%). These results emphasize that both nitrogen-enriched polymers and NH 3 contribute nitrogen atoms together to the highly active sites for the ORR, thus resulting in a high ORR activity. Finally, we constructed a Zn–air battery employing meso/micro-P o PD catalyst loaded on the gas diffusion layer (Teflon-coated carbon fibre paper) as the air cathode and Zn foil as the anode, to demonstrate the potential of our catalyst for real energy devices. Meso-P o PD and the Pt/C catalyst were also tested under the same conditions for comparison. An open-circuit voltage of 1.47–1.50 V was measured for meso-P o PD, meso/micro-P o PD and Pt/C ( Supplementary Fig. 15 ), consistent with the previously reported batteries [13] , [34] . Galvanostatic discharge curves ( Fig. 4a–c ) clearly revealed that the Zn–air battery performance of meso/micro-P o PD electrocatalyst was superior to meso-PoPD and Pt/C with the same catalyst loading, especially at a high current density of 100 mA cm −2 ( Fig. 4c ), and even better than most reported metal-containing catalysts ( Supplementary Table 6 ). The more pronounced advantage of meso/micro-P o PD compared with Pt/C at 100 mA cm −2 was likely because of the hierarchical micro/mesoporous structure that offered mass-transfer benefits at high current densities [11] , [35] . Figure 4: Zn–air battery performance of the catalysts. ( a – c ) Typical galvanostatic discharge curves of Zn–air cells with meso-P o PD, meso/micro-P o PD and Pt/C as cathode catalysts at different current densities: ( a ) 1 mA cm −2 , ( b ) 10 mA cm −2 and ( c ) 100 mA cm −2 . ( d ) Long-time galvanostatic discharge curves of Zn–air cell with meso/micro-P o PD as cathode catalyst until complete consumption of Zn anode. The specific capacity was normalized to the mass of consumed Zn. ( e ) ‘Recharging’ the Zn–air battery with meso/micro-P o PD as cathode catalyst by replenishing Zn anode and electrolyte. Electrolyte for Zn–air cell was 6.0 M KOH. Catalyst loading was 1.0 mg cm −2 for all materials. The arrows indicate ‘recharging’ process. Full size image No obvious voltage drop was observed from the long-term galvanostatic discharge curves until complete consumption of the Zn anode ( Fig. 4d ). Normalized to the mass of consumed Zn, the specific capacity of the Zn–air battery made with meso/micro-P o PD was calculated to be ~630 mAh g −1 , corresponding to gravimetric energy densities of 800 and 630 Wh kg −1 at discharge densities of 10 and 100 mA cm −2 , respectively. After discharging, we found that the battery could be regenerated by refuelling the Zn anode and electrolyte periodically. In such way, the air electrode made with meso/micro-P o PD could work robustly for more than 100 h without any loss of voltage ( Fig. 4e ), highlighting again the high stability of the meso/micro-P o PD catalyst. To summarize, we have demonstrated a fabrication strategy for metal-free ORR electrocatalysts based on the combination of hard-templating synthesis with nitrogen-enriched aromatic polymers as precursors and NH 3 activation. Simultaneous optimization of both porous structure and surface functionality of the nitrogen-doped carbon catalyst was achieved, affording the highest ORR activity (half-wave potential of 0.85 V with a low material loading of 0.1 mg cm −2 ) in alkaline media among all reported metal-free ORR catalysts. More importantly, when used as an ORR catalyst to construct the air electrode for Zn–air battery, our metal-free catalyst outperformed the state-of-the-art Pt/C catalyst. The exceptional ORR activity and durability of our material make it also highly promising as ORR catalyst for other related electrochemical devices, such as alkaline fuel cells [36] , [37] and chlor-alkali electrolysers [38] . We believe that our synthetic protocol for optimizing nitrogen-doped carbonaceous materials can be further extended to fabricate other metal-free and even non-precious metal electrocatalysts with enhanced ORR performance. Moreover, future work will be dedicated to determine the exact structure of active oxygen reduction site of nitrogen-doped carbon catalyst and to better understand the involved reaction mechanism. Electrocatalyst synthesis The fabrication of the meso/micro-P o PD catalyst involves two key steps: (1) hard-templating synthesis; (2) NH 3 activation. For the templating synthesis, briefly, 3.0 g o PD monomer was dissolved in 35 ml 1.0 M HCl and then 22.5 g silica colloid solution (~12 nm, Ludox HS40) was added. After stirring for ~10 min, 12 ml 1.0 M HCl solution containing 7.5 g ammonium peroxydisulphate was added dropwise with vigorous stirring. The polymerization was conducted in an ice bath (<5 °C) for 24 h. After drying the mixture by using a rotary evaporator, the obtained P o PD/Silica composites were pyrolysed under flowing N 2 at 900 °C for 2 h. The silica templates were etched out finally by 2.0 M NaOH to obtain the meso-P o PD. For the NH 3 activation, the prepared meso-P o PD was subjected to a second heat treatment under flowing NH 3 (60 ml min −1 ) at 900 °C for 15 min to form the meso/micro-P o PD. The heating and cooling steps were performed in a N 2 atmosphere. For comparison, p-P o PD with low porosity was prepared by direct pyrolysis of P o PD in the absence of a silica template. A microporous sample (micro-P o PD) was obtained with NH 3 activation of p-P o PD at 900 °C for 15 min. The synthetic protocol was also extended to produce another two porous ORR catalysts, that is, meso/micro-sucrose and meso/micro-PANI, with sucrose and polyaniline as precursors, respectively, through the same hard-templating synthesis/NH 3 activation process. Other activation processes were also employed to prepare porous catalysts based on the meso-P o PD. Meso/micro-PoPD-CO 2 was obtained by activation of meso-P o PD at 900 °C under flowing CO 2 (60 ml min −1 ) for 15 min. Meso/micro-PoPD-KOH was prepared by activation of meso-PoPD with KOH. Briefly, 0.5 g meso-P o PD was mixed with 1.0 g KOH and 10 ml distilled water and stirred for 4 h, followed by another 20 h of static soaking under ambient conditions. After drying at 100 °C, the mixture was heated at 700 °C for 1 h under flowing N 2 . After cooling down naturally, the sample was repeatedly washed by distilled water until a pH value of 7 was reached. The fabrication details and denotation of all samples in this work were summarized in Supplementary Table 1 . Electrochemical measurements All electrochemical measurements were carried out in a conventional three-electrode cell using WaveDriver 20 bipotentiostat (Pine Instrument Company, USA) controlled at room temperature. Ag/AgCl (4 M KCl) and platinum wire were used as reference and counter electrodes, respectively. All potentials in this study refer to that of RHE. The potential difference between Ag/AgCl and RHE is 0.965±0.002 V, based on the calibration measurement in H 2 saturated 0.1 M KOH with polished Pt wires as the working and counter electrodes, and the Ag/AgCl as the reference electrode. A RDE with a glassy carbon disk (5.0 mm diameter) and a RRDE electrode with a Pt ring (6.25 mm inner diameter and 7.92 mm outer diameter) and a glassy carbon disk (5.61 mm diameter) served as the substrate for the working electrodes for evaluating the ORR activity and selectivity of various catalysts, respectively. Before use, the glassy carbon electrodes in RDE/RRDE were polished using aqueous alumina suspensions on felt polishing pads. The catalyst ink was prepared by blending 10 mg catalysts with 100 μl Nafion solution (0.5 wt%) and 0.9 ml ethanol in an ultrasonic bath. A certain volume of catalyst ink was then pipetted on the glassy carbon surface to result in a desirable catalyst loading. RDE/RRDE tests were measured in O 2 -saturated 0.1 M KOH at 1,600 r.p.m. with a sweep rate of 10 mV s −1 . In order to estimate the double layer capacitance, the electrolyte was deaerated by bubbling with argon, and then the voltammogram was evaluated again in the deaerated electrolyte. The oxygen reduction current was taken as the difference between currents measured in the deaerated and oxygen-saturated electrolytes. For detecting peroxide species formed at the disc electrode, the potential of the Pt ring electrode in the RRDE system was set to 1.4 V versus RHE. Commercial 20 wt% platinum on Vulcan carbon black (Pt/C from BASF) was measured for comparison. The working electrode was prepared as follows: 5 mg Pt/C and 50 μl Nafion solution (0.5 wt%) was dispersed in 970 μl of ethanol by sonication for 1 h to obtain a well-dispersed ink. Four microlitres of catalyst ink was then pipetted on the glassy carbon surface, leading to a loading of 0.1 mg cm −2 . Other experimental conditions were the same as for the metal-free catalysts, except that positive scan was recorded for Pt/C to avoid performance loss caused by anions adsorption. The four-electron selectivity of catalysts was evaluated based on the H 2 O 2 yield, calculated from the following equation (1): The electron transfer number can be calculated from the following equation (2): Here, I D and I R are the disk and ring currents, respectively, and N =0.37 is the ring collection efficiency. Zn–air batteries were tested in home-built electrochemical cells, where catalysts loaded on the gas diffusion layer (Teflon-coated carbon fibre paper, 1.0 cm 2 , catalyst loading 1.0 mg for all materials) as the air cathode and Zn foil as anode in 6.0 M KOH. Measurements were carried out on the as-fabricated cell at room temperature with a CHI 760E (CH Instrument, USA) electrochemical workstation. Characterization TEM was performed using a JEM-1400 (JEOL Ltd, Japan) operating at an accelerating voltage of 200 kV. X-ray photoelectron spectroscopy experiments were carried out on an AXIS Ultra DLD system from Kratos with Al Kα radiation as X-ray source for radiation. Nitrogen sorption isotherms were measured at 77 K on ASAP 2020 and TriStar 3020 volumetric analyzers (Micromeritics, nc., GA). Before measurements, all samples were degassed at 300 °C for at least 3 h. The specific surface area was determined by standard BET method in the relative pressure range of 0.05–0.2. The PSD curves were calculated by the nonlocal density functional theory in the range up to 2 nm, and by the Barrett–Joyner–Halenda method in the range of 2~100 nm. How to cite this article : Liang, H.-W. et al. Hierarchically porous carbons with optimized nitrogen doping as highly active electrocatalysts for oxygen reduction. Nat. Commun. 5:4973 doi: 10.1038/ncomms5973 (2014).